Locating and classifying fluorescent tags behind turbid layers using time-resolved inversion The use of fluorescent probes and the recovery of their lifetimes allow for significant advances in many imaging systems, in particular, medical imaging systems. Here we propose and experimentally demonstrate reconstructing the locations and lifetimes of fluorescent markers hidden behind a turbid layer. This opens the door to various applications for non-invasive diagnosis, analysis, flowmetry and inspection. The method is based on a time-resolved measurement that captures information about both fluorescence lifetime and spatial position of the probes. To reconstruct the scene, the method relies on a sparse optimization framework to invert time-resolved measurements. This wide-angle technique does not rely on coherence, and does not require the probes to be directly in line of sight of the camera, making it potentially suitable for long-range imaging. With the ability to control and manipulate luminescent probes, fluorescence imaging has become a major workhorse in many imaging systems. Besides providing high-resolution results in biological microscopy [1] , [2] , fluorescence imaging has been found useful in many other applications, including the study of turbulence [3] , [4] and high-temperature reactions [5] , the production of optical tags for anti-fraud measures or covert tracking [6] , and the remote sensing of vegetation [7] . These radiance measurements are further supplemented with fluorescence lifetime imaging (FLI) data. Though it requires more complex hardware, FLI provides great detail about the environment of the probes, including mixing dynamics [8] and energy transfer mechanisms [9] , and it resolves ambiguous spectral radiance measurements by unmixing multiple fluorescence markers and auto-fluorescence [10] . Time-resolved FLI is useful for fluorescence localization in turbid media using asymptotic decay approximations [11] and early photons [12] , [13] , [14] , with hybrid models under study [15] . Though fluorescence decay broadens the pulse duration, early-photon FLI measurements can still localize objects using the relatively fast rise time [16] , [17] . This high-frequency temporal structure competes with the low-frequency decay. Therefore, in an imaging modality, a time-resolved image that is high-pass temporally filtered should reveal these edges, which in turn contain information about the spatial configuration of the fluorescent markers. However, typical imaging systems use either widefield gated intensified charge-coupled device cameras (time resolution ∼ 100s ps) or fiber-coupled sensors, and have not made full use of the spatial variation of early photons and fluorescence lifetime simultaneously. Here we propose and demonstrate a three-dimensional widefield time-resolved method for locating fluorescent probes through diffuse layers by looking only at a single one-dimensional (1D) horizontal line on the diffuser. We overcome the inherent temporal blurring due to long fluorescence decay times by using a sparse optimization. Thus, the method is a two-step process: (1) record the time-resolved scattering of fluorescent markers; and (2) use prior knowledge of the scene to recover the positions of the fluorescent markers and classify them via their lifetimes. Because of the inherent wide-angle field of view of our time-resolved technique [18] , [19] , the method has potential use in areas such as long-range imaging through turbulence and widefield tomography using early-photon arrival times. The integration of a sparse prior here allows for recovering object information in the presence of long lifetimes. Previous methods [18] , [19] require the high temporal resolution and would fail to recover nanosecond emission. The suggested method does not require the fluorophore to be directly in the field of view of the camera. Instead the tags can be localized and identified as long as the photons from the fluorescent emission of the tags can reach the camera lens in the recorded time window. The technique is implemented non-invasively in reflective mode. This opens a new set of possibilities for applications such as tracking and locating probes in photocytometry [20] , endoscopy [21] and larger-scale industrial tomography [22] . Forward model Consider the sketch shown in Fig. 1a . Laser light (L) scatters through a diffuse layer (D) towards an object (O), which produces some response R . Light then scatters back towards the diffuser and is imaged onto a time-resolved sensor (C). 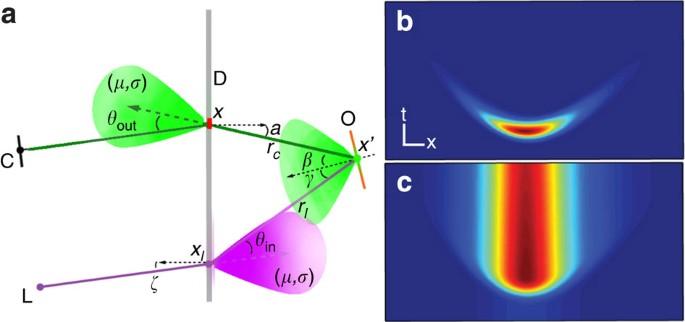Figure 1: Measurement geometry and output streak images. (a) Geometry of diffuser and patch. (b) Example of recorded streak image for a non-fluorescing patch, that is,τ→0 and (c) for a fluorescing patch withτ=5 ns. Scale bars, 100 ps (vertical), 1 cm (horizontal). For a given incident laser pulse at position x l with incident power of I 0 , the measured time-resolved image is given by [18] , [19] Figure 1: Measurement geometry and output streak images. ( a ) Geometry of diffuser and patch. ( b ) Example of recorded streak image for a non-fluorescing patch, that is, τ →0 and ( c ) for a fluorescing patch with τ =5 ns. Scale bars, 100 ps (vertical), 1 cm (horizontal). Full size image where * t denotes convolution in time, r l ( x′ ) =||x′−x l ||, r c ( x′ ) =||x′−x|| , and g ( x l , x , x′ ) is a time-independent physical factor that depends on the system geometry: The angles { α , β , γ , ζ , θ in/out } are defined by the geometry in Fig. 1a . N ( θ ) is the diffuser scattering profile, characterized by a scattering width σ . For the 0.7-mm-thick polycarbonate diffuser considered here, N is Gaussian: N ( θ )=exp( −θ 2 /2 σ 2 ), with σ ≈60°. The object response function R is generally a function of the reflectance (including, for example, the efficiency) of an object point, as well as a function of time. For fluorescent markers, the lifetime and efficiency can vary in space. Here each point in the object volume can contain a single but different exponential decay: where ρ ( x′ ) is the local time-independent reflectance, τ ( x′ ) is the local lifetime and u ( t ) is the unit step function imposed to satisfy causality constraints. Note that the delta function confines intensity to a hyperbolic path in the x–t plane: a streak image for a single-point source (ignoring any time response in R ) is a hyperbola. For a single-shot image acquisition system, equation (1) is the recorded time-resolved image. However, for a pulse train (which is used experimentally to increase signal-to-noise ratio (SNR)), the fluorescent lifetimes must be compared with the repetition rate T of the illumination. If τ ∼ T , then the fluorescent decay from the current pulse is superposed with the decays from previous pulses. Quantitatively, if we model the illumination with a pulse train, the streak image becomes Substituting equation (3) into equation (4), we have (see Supplementary Note 1 ) where is the integer floor function. Here we assume that there is only a small number of fluorescent particles in the field of view. Thus, we measure the fluorescence dynamics of discrete object points, located at coordinates x j with lifetime τ j : A simulated time-resolved measurement for a non-fluorescent and a fluorescent point object is shown in Fig. 1b and Fig. 1c , respectively. Equation (6) is a time-periodic function. To gain some intuition, we ignore all spatial dependence and focus on the time dependence, plotted in Fig. 2 for a single fluorescent point. 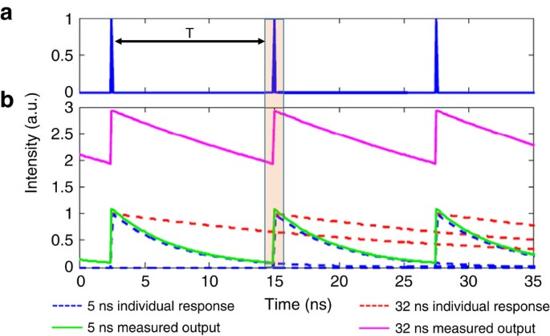Figure 2: Time-resolved fluorescence imaging with a pulse train. (a) Incident pulse train, separated by periodT. (b) Measured output for a fluorescent marker with lifetimes 5 and 32 ns. Dashed lines indicate the individual response for a single pulse. Solid lines indicate the measured signal. The orange box indicates detector time window. Figure 2a shows the incident pulse train with repetition rate T . Compared with all other temporal parameters, the pulse duration can be considered negligible. Figure 2b shows the time response for τ/T= 0.40 and τ/T= 2.56, respectively. The dashed curves represent the individual responses due to each pulse and the solid curves represent the expected measurement. We see that for longer lifetimes, the contrast of the measured signal decreases due to the residual fluorescence from previous pulses. If we define the contrast V as the difference between the maximum and minimum intensity values divided by the sum, we find that V= tanh ( T/ 2 τ ) (see Supplementary Note 1 ). Longer lifetimes, therefore, tend to increase the ‘dc’ component of the signal relative to the high-frequency edges. This is effectively a low-pass filtering operation in time. Therefore, previous methods [18] , [19] for reconstructing objects in similar environments must be modified. Figure 2: Time-resolved fluorescence imaging with a pulse train. ( a ) Incident pulse train, separated by period T . ( b ) Measured output for a fluorescent marker with lifetimes 5 and 32 ns. Dashed lines indicate the individual response for a single pulse. Solid lines indicate the measured signal. The orange box indicates detector time window. Full size image We seek to answer the following question: given a set of time-resolved measurements { I l } ( l= 0,1,..., L ), what are the locations ( x j ) and lifetimes ( τ j ) of the fluorescent tags generating the signal? A sparsity constraint allows us to separate the problem into two steps (see Reconstruction algorithm subsection below) and to overcome strong signal overlap. Note that this is the physical insight for subwavelength resolution using PALM or STORM microscopy [23] , [24] and single-pixel acquisition modalities [25] . Our extensions here offer similar possibilities in remote sensing. Reconstruction algorithm To recover the unkown positions and lifetimes from a set of time-resolved measurements, we separate the problem into two steps. We first recover the objects’ positions. Then, using the measurmenents and recovered positions, we classify the objects via lifetimes. The reconstruction flow is shown in Fig. 3 . This two-step process allows us to exploit the sparsity of the geometry information by avoiding the signal overlap due to relatively long fluorecence decay times. 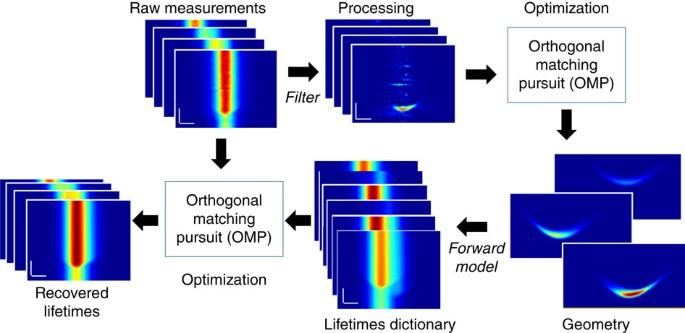Figure 3: Reconstruction flow. Raw measurements are filtered to produce streak hyperbolas; geometry is recovered via OMP; a lifetime dictionary is created; and another OMP step identifies lifetimes of the probes. Figure 3: Reconstruction flow. Raw measurements are filtered to produce streak hyperbolas; geometry is recovered via OMP; a lifetime dictionary is created; and another OMP step identifies lifetimes of the probes. Full size image At the first step, we aim to localize the patches. Ideally, the data could be deconvolved with an appropriate R ( x , t ), but we do not know the individual lifetimes in advance. Instead, we operate on each streak image a simple high-pass temporal filter (first-order derivative) and zero all resulting negative values. The result is a set of streak images { I l ( F ) } that contain (approximately) only the edge structures, and hence geometrical information. We then define a measurement Ī l to be the vectorized form of a single time-resolved image I l ( F ) , that is, Ī l is an MN × 1 vector. We concatenate all L vectors into a single LMN × 1 data vector: I meas =( Ī 1 T Ī 2 T … Ī L T ) T . This is a complete experimental measurement. Next, we define a vector I p as the expected data from a single non-fluorescent object located at point x p . We can create a dictionary matrix D whose columns consist of the expected data of all possible point locations and lifetimes: D =( I 1 I 2 ... I P ). Thus, for a set of object points with weights ρ , we can write the system in a vector-matrix form as where the elements of ρ =( ρ 1 ρ 2 ... ρ P ) T are the reflectance values of each potential object point (0< ρ p <1). Note that if the number of object points in the experiment is much less than the total length of ρ , then most elements of ρ are zero. Thus, we can recover the non-zero elements of this vector using a sparsity-promoting algorithm. The positions of each non-zero element determine the location of the object points. We seek to solve the following optimization problem: where the l 0 norm equals the number of non-zero elements in ρ , and ɛ represents an error tolerance due to noise. To build the dictionary matrix D , we simulate (via equation 1) the expected streak images for a single patch and computationally scan its location throughout the working volume. Equation (8) is solved via orthogonal matching pursuit (OMP) [26] to yield the dictionary atoms (or unit cells) that are best correlated with the filtered streak images. OMP is a greedy algorithm, which searches sequentially for the best atom that matches the input, subtracts its contribution from the data and iterates this process until the residual error derivative is below a user-defined threshold. The number of iterations equals the number of objects recovered. With the locations of all patches recovered in the first step, we move onto the second step and render all possible florescent images using a known set of potential lifetimes. For N p patches and N f potential lifetimes, there are N p N f atoms in this new fluorescent dictionary. The fluorescent dictionary and the measured (unfiltered) fluorescent data are input into another OMP iteration with the residual error derivative as a stopping criterion. The lifetimes are also recovered in this process. We note that due to the noisy input to the OMP algorithm from step 1, we usually recover too many patches (relaxed stopping criterion, see Supplementary Note 2 ); however, these are always removed in the second step and the correct number of patches is recovered. Experimental demonstration The scene is a set of three 1.5 × 1.5 cm 2 square patches ( Fig. 4a,b ) hidden behind a diffuser. The first patch (NF) is non-fluorescent. The second patch (QD) is painted with a quantum dot solution ( τ =32 ns, λ emission ∼ 652 nm; ref. 27 ). The third patch (PI) is painted with Pyranine ink ( τ= 5 ns, λ emission ∼ 510 nm; ref. 28 ). 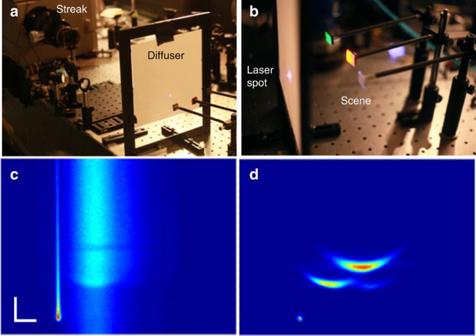Figure 4: Experimental geometry and streak images. (a) Experimental set-up. (b) Scene under investigation. (c) Sample FLI measurement with decay times extending throughout the entire image. (d) Non-fluorescent analogue of (c) (recorded without ultraviolet filter). The diffuser is fluorescent, noted by the decay of the calibration spot in (c). Scale bars, 4.2 cm (horizontal), 200 ps (vertical). Figure 4: Experimental geometry and streak images. ( a ) Experimental set-up. ( b ) Scene under investigation. ( c ) Sample FLI measurement with decay times extending throughout the entire image. ( d ) Non-fluorescent analogue of ( c ) (recorded without ultraviolet filter). The diffuser is fluorescent, noted by the decay of the calibration spot in ( c ). Scale bars, 4.2 cm (horizontal), 200 ps (vertical). Full size image We carry out three experiments, each with a different patch configuration. Each column in Fig. 5 corresponds to a different configuration. 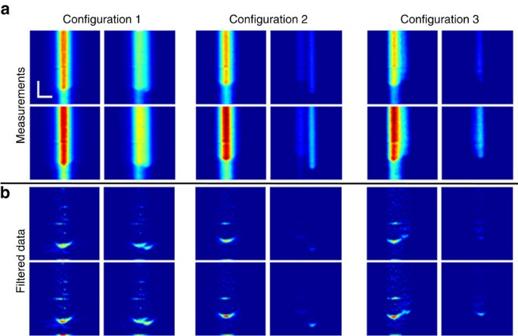Figure 5: Experimental measurements as input to the algorithm. Each column is a different configuration, and for each we show (a) example of four measurements taken and (b) the corresponding high-pass filtered images. Scale bars, 4.2 cm (horizontal), 200 ps (vertical). The four points correspond to measurements with illumination positions x12, x11, x9and x8as shown by the labels inFig. 10. Figure 5a shows the experimental measurments. For each configuration, we input the filtered data ( Fig. 5b ) into OMP to recover the location of each patch. After reconstructing the lifetimes, we use the forward model (equation 6) to generate streak images that match the measurments ( Fig. 6a ). The reconstructions are shown in Fig. 6b . Because we use an ultraviolet filter, no information from the NF patch is recorded. We note that the fluorescent lifetimes are always identified correctly, and that the position error is on the order of the patch size or dictionary resolution ( Table 1 ). Finally, because we assume only a finite number of lifetimes, the algorithm distinguishes between the PI and QD patches with no errors. We emphasize here that the reconstruction is spectrally invariant, so that two patches with the same emission wavelength can still be separated. Figure 5: Experimental measurements as input to the algorithm. Each column is a different configuration, and for each we show ( a ) example of four measurements taken and ( b ) the corresponding high-pass filtered images. Scale bars, 4.2 cm (horizontal), 200 ps (vertical). The four points correspond to measurements with illumination positions x 12 , x 11 , x 9 and x 8 as shown by the labels in Fig. 10 . 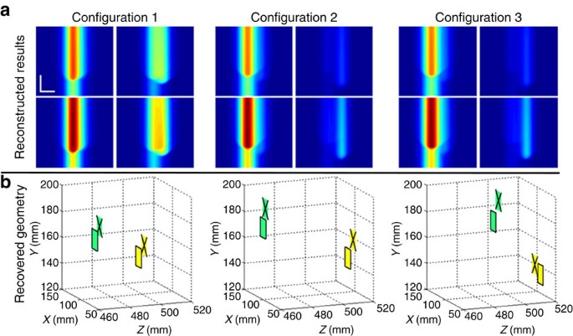Figure 6: Reconstruction results. (a) Reconstructed streak images using the recovered locations and lifetimes. Scale bars, 4.2 cm (horizontal), 200 ps (vertical). (b) Geometry recovered for each configuration. Green and yellow correspond to PI and QD patches, respectively. Patches with anXare the recovered locations; solid outlines indicate ground truth (measured by a Faro Gage Arm). The four points correspond to measurements with illumination positions x12, x11, x9and x8as shown by the labels inFig. 10. Full size image Figure 6: Reconstruction results. ( a ) Reconstructed streak images using the recovered locations and lifetimes. Scale bars, 4.2 cm (horizontal), 200 ps (vertical). ( b ) Geometry recovered for each configuration. Green and yellow correspond to PI and QD patches, respectively. Patches with an X are the recovered locations; solid outlines indicate ground truth (measured by a Faro Gage Arm). The four points correspond to measurements with illumination positions x 12 , x 11 , x 9 and x 8 as shown by the labels in Fig. 10 . Full size image Table 1 Reconstruction error; the numbers represent distances from the centre of each ground truth patch in space to the centre of the corresponding reconstructed patch (length units are millimetres). Full size table Currently, we are modelling turbulence by scattering layers. This is common [29] , but can be extended beyond to thick media, provided the temporal blurring due to multiple scattering still allows us to resolve the fluorescence rise time via filtering [19] . Theoretically, there is no fundamental limit precluding the extension of our method to volume scattering. The main issues are practical, namely, a reduction in SNR with an increase in complexity in forward modelling. However, the sparse prior we exploit here can alleviate these constraints. Since fluorescence signals are commonly sparse in nature, sparsity is a natural way to avoid local minima during reconstruction (as would occur in standard optimization methods) and to achieve a robust solution relatively quickly (that is, in minutes rather than days). It is specifically the sparse prior that allows reconstruction in the presence of long lifetimes over narrow time windows. We provide detailed comparison of our method with other techniques in Supplementary Note 3 ; our system offers wider field of view [30] and does not rely on coherence [31] , [32] . With our method, the relevant parameters are the diffusion constant, thickness of the diffuser and the system time resolution. Because the illumination intensity at the excitation wavelength is stronger than the emission, without an ultraviolet filter we can filter out the fluorescence and use only the geometrical information (including non-fluorescent objects) in the first OMP step. This results in higher reconstruction accuracy, but requires twice the recording time. Ultimately, however, the underlying limits of the system are SNR and the accessible volume. One straightforward way to alleviate this for a remote sensing application is to increase the laser power. This can be done provided it is not harmful to the targets under study, so it is preferable to use the minimum laser power (lowest SNR) that still enables correct reconstruction. In our system, changes in the patch size behind the diffuser affect the peak SNR (PSNR) as in Fig. 7 . The red markers are measured data and the blue curve is the result of our forward model. For each image we estimate the noise by using the algorithm described in ref. 33 . While the signal strength increases with the patch size, the estimated noise levels in all five measurements are identical (within 1.5% of the noise mean). As expected the PSNR improves for larger patches. Note that the measured PSNR of the largest patch is slightly lower than what is expected from the forward model; this can be explained by nonlinear behaviour of the streak tube dynamic range near the saturation level of the sensor. 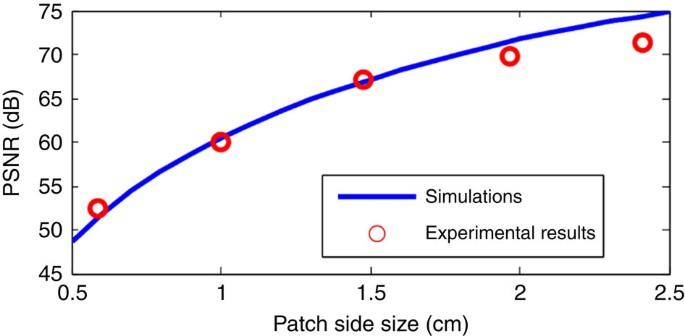Figure 7: Patch size effect on PSNR. The red dots are experimental measurements (taken with fixed exposure and gain) and the blue curve is a forward model simulation prediction (we add to simulated measurements white Gaussian noise with variance that matches the measured variance). Figure 7: Patch size effect on PSNR. The red dots are experimental measurements (taken with fixed exposure and gain) and the blue curve is a forward model simulation prediction (we add to simulated measurements white Gaussian noise with variance that matches the measured variance). Full size image On the basis of the effect of patch size on PSNR, the reconstruction error is also indirectly a function of patch size. To understand the effects of noise, we analyse the reconstruction accuracy as a function of measurement noise and patch size ( Fig. 8 ). Twelve time-resolved images are simulated (via equation (1)) using three different fluorescent objects, with white Gaussian noise added to the images. These images are then input into the reconstruction algorithm. 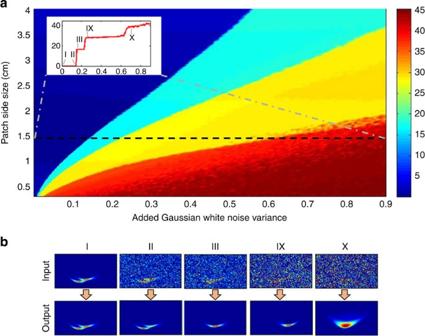Figure 8: Noise performance. (a) Analysis of reconstruction error as function of patch side size and added noise. White Gaussian noise with increasing variance (x-axis) is added while increasing the patch’s size (y-axis). The colour represents the total algorithm reconstruction error in arbitrary units. Inset figure shows the algorithm sensitivity along the black dashed line (corresponding to patch size of 1.5 cm). (b) Examples of different points on the inset graph that show input images with added noise and the reconstruction results. These images correspond to one of the twelve illumination points. Figure 8a shows the reconstruction error as a function of the noise level and patch size. The plotted error is a sum of all three distances between the reconstructed objects and the corresponding ground truth locations of fluorescing patches divided by the diagonal size of dictionary voxel. The error results show three step-like changes for all patch sizes ( Fig. 8a ); as the patch size increases the signal level increases, and the first jump in error is postponed to larger added noise. It should be noted that for all simulations, we used the original dictionary designed for 1.5 × 1.5 cm patches. Figure 8: Noise performance. ( a ) Analysis of reconstruction error as function of patch side size and added noise. White Gaussian noise with increasing variance ( x -axis) is added while increasing the patch’s size ( y -axis). The colour represents the total algorithm reconstruction error in arbitrary units. Inset figure shows the algorithm sensitivity along the black dashed line (corresponding to patch size of 1.5 cm). ( b ) Examples of different points on the inset graph that show input images with added noise and the reconstruction results. These images correspond to one of the twelve illumination points. Full size image We see that for low noise variance, the error is virtually zero. As the noise increases, step-like jumps in the error are noted. At first, this seems counter-intuitive: we expect the error to increase continuously with noise. However, the discontinuities occur as a result of the sparsity-based method. At specific noise levels, OMP cannot distinguish between different curves, and so an atom is essentially lost ( Fig. 8 ). This occurs at thresholds when the energy of the lost atom is comparable to the noise level. After this threshold, the algorithm selects a different (incorrect) atom that overlaps with one of the remaining, stronger atoms (transitions from II to III and from III to IX). When the last atom is lost (point X), the algorithm chooses the atoms with the largest foot print. Similar analysis for choosing the patches’ lifetimes showed that the lifetime estimation is even more robust to noise. As seen from the reconstructions presented in Fig. 6 , the patches are not required to be directly in the line of sight of the camera; therefore, unlike a conventional imaging system with a field of view, we need to define an accessible volume (or visible volume) for this imaging system ( Fig. 9a,b ). Because there are two sequential scattering events before the signal reaches back to the diffuser, the detected signal must fall off as the product of the square of the distances r c and r l . Assuming r c ≈r l =r , we have I l ∼ I 0 /r 4 (equations 1 and 2). Therefore, a larger accessible volume is obtained at the expense of lower SNR. The intensity contrast from the closest object point ( r D 1 ) to the farthest point ( r D 2 ) should be within the dynamic range of the camera to avoid saturation, and the signal from the farthest point must be above the noise floor. 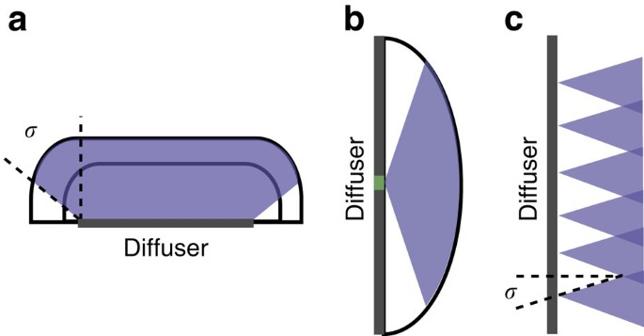Figure 9: Visible volume. (a) Top and (b) side views of visible volume. The inner black curve shows the saturation bound and the outer black curve shows the noise-limited bound. The purple area shows the geometry limitation imposed by diffusion/scattering angles (σ). The green rectangle in the middle of the diffuser is the line imaged by the camera (conventional field of view). (c) Illumination gaps due to small scattering angles and widely spaced illumination points. We can write these conditions as: Figure 9: Visible volume. ( a ) Top and ( b ) side views of visible volume. The inner black curve shows the saturation bound and the outer black curve shows the noise-limited bound. The purple area shows the geometry limitation imposed by diffusion/scattering angles ( σ ). The green rectangle in the middle of the diffuser is the line imaged by the camera (conventional field of view). ( c ) Illumination gaps due to small scattering angles and widely spaced illumination points. Full size image where K is a constant that is inversely proportional to σ (the scattering angle of the diffusive layer). Combining equations (9) and (10), we find that the maximum and minimum distances are r D 2 =( KI 0 /I noise ) 1/4 and r D 1 =( KI 0 /I sat ) 1/4 . This gives us the intensity constraints on the maximum potential accessible volume ( Fig. 9a,b ). Further, the scattered light from all points must arrive within the sensor’s time window T w : ( r c +r l ) max − ( r c +r l ) min ≤cT w . Thus, for a given incident laser position x l , the accessible volume is the intersection of the volumes given by this time constraint and the intensity constraints ( Fig. 9b ). Note also that this volume is trimmed if σ is <90°. Finally, the number of illumination points L controls the total visible volume, which is the concatenation of L volumes described above for each laser position x l . Further, for a scattering angle <90°, there can be gaps in the accessible volume close to the diffuser ( Fig. 9c ). Overall, increased scattering increases the accessible volume close to the diffuser. Therefore, the ability to reconstruct images is thus a competition between SNR, which is reduced by scattering, and the accessible volume, which is enhanced by it. In summary, we demonstrated time-resolved inversion of scattered light to locate fluorescent tags behind diffusive layers in wide-angle scenes and to identify their lifetimes. This technique, which relies on sparse optimization, has potential applications in remote sensing of spectrally identical fluorescent tags and offers algorithmic benefits for fluorescence lifetime tomography beyond the conventional line of sight of the camera. Optical set-up The experimental set-up is shown in Fig. 10 and Fig. 4a,b . A Titanium:Sapphire laser (1.15 W ( ∼ 15 nJ per pulse), λ= 800 nm, T= 12.5 ns repitition rate and 50 fs pulse duration) is frequency doubled using a barium borate crystal to 400 nm and is then focused ( ∼ 100 mW average power at the focus) onto a polycarbonate diffuser (Edmund Optics, 55–444) with a scattering angle of ∼ 60°. Light is scattered towards a scene, which scatters light back towards the diffuser, the front side of which is imaged onto a streak camera (Hamamatsu C5680) with a time resolution of 2 ps and a time window of 1 ns. The detector has a 1D aperture and records the time profile of a horizontal slice of the diffuser, with an x–t resolution of M × N =672 × 512 pixels. To increase SNR, the total exposure time is T int =10 ms, so that a given streak image integrates light scattered from T int /T incident pulses. Because the streak camera has only a 1D horizontal aperture, we scan the incident laser position across L= 12 positions to mimic a two-dimensional aperture [34] and record 12 streak images. The total acquisition time is approximately LT int . 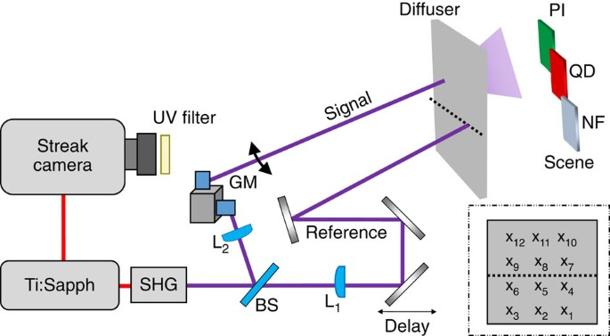Figure 10: Experimental set-up. A 1.15 W Ti:Sapphire beam is frequency doubled and is focused onto a diffuser via a pair of galvo mirrors (GM), which scan the beam across the diffuser to different incident positions (inset). Light is scattered by various objects and is recorded by a streak camera (field of view indicated by the dotted line). A fixed reference beam is used to correct for intensity and timing noise. Inset: locations of incident laser positions for each streak image. Figure 10: Experimental set-up. A 1.15 W Ti:Sapphire beam is frequency doubled and is focused onto a diffuser via a pair of galvo mirrors (GM), which scan the beam across the diffuser to different incident positions (inset). Light is scattered by various objects and is recorded by a streak camera (field of view indicated by the dotted line). A fixed reference beam is used to correct for intensity and timing noise. Inset: locations of incident laser positions for each streak image. Full size image To calibrate intensity fluctuations and temporal jitter, a portion of the incident laser beam is split off and focused onto the diffuser, directly in the view line of the camera, so that a streak image of a direct reflection is observed. This calibration spot is fixed for the duration of the acquisition of all streak images (incident laser positions) and is used to subtract any timing jitter noise in the detector and to scale any intensity fluctuations. The calibration point is then cropped to reduce errors during the reconstruction process. Fluorescent marker parameters The scene is a set of three 1.5 × 1.5 cm 2 square patches ( Fig. 4b ). The first patch (NF) is non-fluorescent, cut from a white MacBeth Colorchecker square. The second patch (QD) is painted with a CdSe-CdS quantum dot solution ( τ =32 ns, λ emission ∼ 652 nm; ref. 27 ). The third patch (PI) is painted with Pyranine ink ( τ= 5 ns, λ emission ∼ 510 nm; ref. 28 ). To study the time-resolved scattering of both the ultraviolet excitation (400 nm) and the fluorescent emission (652 nm from QD and 510 nm from PI), images are recorded both with and without an ultraviolet cutoff filter ( λ cut =450 nm). The ultraviolet filter eliminates the ultraviolet reflection from the patches and with it, only the visible fluorescence emission profile is captured by the camera (for example, Fig. 4c ). A non-fluorescent analogue is shown in Fig. 4d . Only the images taken with the ultraviolet cutoff filter are used for reconstruction, thus information for the NF patch is not measured. While each of these probes has several main absorption bands, the closest dominant absorption maxima for QD and PI are at 600 and 460 nm, respectively [27] , [35] . Therefore, 400-nm illumination can properly excite the probes into fluorescent mode. Algorithm parameters The geometry dictionary resolution is chosen to be dx=6.9 mm, dy=7.5 mm and dz=5.2 mm. The volume of interest results in 18,856 atoms in the dictionary. Therefore, using the full-resolution streak images results in a vector of size 12 × 512 × 672=4,128,768. Storing the full dictionary requires approximately 622 GB of memory. By down-sampling each image to 51 × 67 pixels, a vector length of 41,004 is obtained for the 12 images, which results in dictionary size of 6.2 GB. This is a factor of 100 reduction in computational burden. Another approach that might be considered is the use of sparse representation; however, since the dictionary structure is highly irregular, this approach is not beneficial. The lifetime dictionary is far smaller than the geometry dictionary, which allows us to use full-resolution images. Using an unoptimized MATLAB code and a desktop computer (Intel Core i7 with 32 GB RAM), it took the algorithm 91 s per reconstruction on average. How to cite this article: Satat, G. et al . Locating and classifying fluorescent tags behind turbid layers using time-resolved inversion. Nat. Commun . 6:6796 doi: 10.1038/ncomms7796 (2015).